Production of α-L-iduronidase in maize for the potential treatment of a human lysosomal storage disease Lysosomal storage diseases are a class of over 70 rare genetic diseases that are amenable to enzyme replacement therapy. Towards developing a plant-based enzyme replacement therapeutic for the lysosomal storage disease mucopolysaccharidosis I, here we expressed α- L -iduronidase in the endosperm of maize seeds by a previously uncharacterized mRNA-targeting-based mechanism. Immunolocalization, cellular fractionation and in situ RT–PCR demonstrate that the α- L -iduronidase protein and mRNA are targeted to endoplasmic reticulum (ER)-derived protein bodies and to protein body–ER regions, respectively, using regulatory (5′- and 3′-UTR) and signal-peptide coding sequences from the γ-zein gene. The maize α- L -iduronidase exhibits high activity, contains high-mannose N-glycans and is amenable to in vitro phosphorylation. This mRNA-based strategy is of widespread importance as plant N-glycan maturation is controlled and the therapeutic protein is generated in a native form. For our target enzyme, the N-glycan structures are appropriate for downstream processing, a prerequisite for its potential as a therapeutic protein. Lysosomal storage diseases (LSDs) are a broad class of genetic diseases that are caused by mutations in proteins critical for lysosomal function; collectively, they represent over 70 disorders [1] , [2] , [3] , [4] , [5] . In many of these diseases, there is a deficiency of a single hydrolase enzyme within the lysosome; all are progressive in nature, as the affected individual is unable to degrade certain macromolecules, a process essential for normal growth and homeostasis of tissues. Many LSDs are amenable to enzyme replacement therapy (ERT)—a process that takes advantage of plasma membrane receptor mechanisms that mediate cellular uptake of a recombinant purified enzyme following its intravenous delivery [6] . ERT has become established for six of the LSDs. One of the mucopolysaccharidoses, MPS I, is an LSD characterized by the deficiency of α- L -iduronidase, an enzyme involved in the stepwise degradation of glycosaminoglycans; in severely affected humans, this genetic disease is characterized by profound skeletal, cardiac, and neurological pathology and death in early childhood [7] . The average annual costs of the ERT drug for MPS I disease (Laronidase or Aldurazyme) range from $300,000 USD (children) to $800,000 USD (adults). Transgenic plants, cultured plant cells and seeds are potentially cost-effective and safe systems for large-scale production of recombinant therapeutic proteins; they offer considerable advantages as production systems, but are not without challenges [8] , [9] . The majority of human lysosomal enzymes are glycoproteins and the nature of their N-glycan structures can influence their stability, transport and biological activity. Within the Golgi complex of both plant and animal cells, enzymes convert many of the original high-mannose N-glycans of proteins to complex N-glycans through sequential reactions that rely on accessibility of the glycan chain(s) to the Golgi-processing machinery [9] , [10] . In the mammalian Golgi complex, many of the N-glycan core structures (Man 3 GlcNAc 2 ) are extended further to contain penultimate galactose and terminal sialic acid residues [10] . In contrast, typically processed N-linked glycans of plant proteins are mostly of a Man 3 GlcNAc 2 structure with or without β-1,2-xylose and/or α-1,3-fucose [9] . For glycoprotein therapeutics destined for parenteral administration (as in ERT), the presence of plant-specific xylose and/or fucose residues is problematic, because the therapeutic is potentially highly immunogenic [9] . Different strategies have been used to modify the N-glycan processing of plant-made recombinant proteins; one strategy has been to manipulate subcellular protein targeting to avoid Golgi transport [8] , [9] . This has involved the addition of C-terminal HDEL/KDEL sequences or similar motifs for endoplasmic reticulum (ER) retention, or the addition of transmembrane and cytoplasmic tail sequences that potentially act as anchors for delivering recombinant proteins to vacuolar compartments independent of the Golgi complex [11] . These strategies suffer the drawbacks of requiring the addition of foreign amino acids that remain on the mature recombinant protein. The HDEL/KDEL strategy is very efficient for controlling the N-glycosylation of some recombinant proteins, especially antibodies [12] , [13] , [14] . However, the efficacy of this strategy is protein-specific [9] . For some recombinant proteins, including human α- L -iduronidase produced in Arabidopsis seeds, there is clearly an insufficient control of N-glycan maturation [15] . The use of vacuolar anchors as a means of controlling complex N-glycan formation [11] is not yet backed up by definitive evidence. The mechanisms by which proteins of eukaryotic cells are targeted intracellularly are most commonly mediated through signals on the protein itself (for example, amino acid or carbohydrate motifs). More recently, it has been recognized that signals on mRNAs can also mediate the targeting of proteins to specific intracellular regions [16] , [17] . γ-Zein storage proteins (prolamins) of maize seeds are deposited in ER-derived protein bodies and do not transit through the Golgi complex [18] . In the present study, we exploited the potential of maize seeds for hosting the production of recombinant human α- L -iduronidase by taking advantage of their capacity for ER–protein body localization of the gene product. We hypothesized that α- L -iduronidase would be targeted to ER-derived protein bodies by mRNA targeting using γ-zein cis -elements. If successful, the 'native' recombinant therapeutic protein (that is, possessing no foreign amino acid motifs) would stably accumulate in maize endosperm cells, but have avoided transit through the Golgi complex and the consequent undesired N-glycan maturation. We found that the regulatory (5′- and 3′-untranslated region (UTR)) and signal-peptide-encoding sequences of the γ-zein gene are sufficient for direct ER–protein body deposition of the majority of the α- L -iduronidase by an mRNA-targeting-based mechanism. Moreover, the α- L -iduronidase was enzymatically active and possessed kinetic characteristics that were comparable to those of the commercial MPS I ERT product (Aldurazyme). After immunoadsorbing the minor contaminant of Golgi-modified enzyme, the affinity-purified maize recombinant α- L -iduronidase contained exclusively high-mannose N-glycans and was amenable to in vitro phosphorylation using a recombinant soluble GlcNAc-1-phosphotransferase, which is the first step to creating the mannose-6-phosphate (M6P) lysosomal sorting motif. We discuss the widespread importance of the targeting of recombinant proteins to ER-derived protein bodies in maize by mRNA targeting for therapeutic protein production. Importantly, no topogenic information from mature-protein-coding sequences of γ-zein was required to accumulate the human recombinant protein; hence, the production mechanism avoids the requirement of engineering a proteolytic cleavage site for removal of non-native amino acids. Strategy for expression of human α- L -iduronidase in maize To investigate the capacity of an mRNA targeting mechanism to direct the localized accumulation of our recombinant human enzyme in maize seeds, we designed two constructs—a test construct containing the putative cis mRNA-targeting elements of the 27-kDa γ-zein gene and a control construct with substituted sequences ( Fig. 1a,b ). The test construct contained the 71-bp 5′-UTR, signal peptide-encoding sequences and the 3′-UTR terminator, all from the γ-zein gene. As with the test construct, the control construct contained the γ-zein promoter and 62 bp of the γ-zein gene 5′-UTR, but in contrast, contained 10 bp of 5′-UTR and signal peptide-encoding sequences of the α- L -iduronidase gene; the 3′-region was derived from the Nos ( nopaline synthase ) gene. 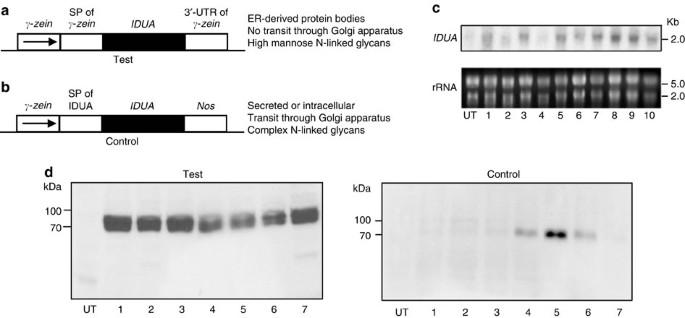Figure 1: Constructs and expression of recombinant human α-L-iduronidase in transgenic maize. Gene constructs for expression in maize seeds and the predicted glycosylation status and subcellular localization of the synthesized protein derived from expression of these constructs (a,b).Nos,nopaline synthase(Nos) gene 3′-region; SP, signal peptide; 3′-UTR, 3′-untranslated region. The humanα-L-iduronidase(IDUA) gene was driven by the 1638-bpγ-zeinpromoter (constructs shown ina,b). Additionalγ-zeingene regulatory sequences flanking theα-L-iduronidasemature coding region included the 71-bp 5′-UTR, the signal peptide-encoding sequences (57 bp) and the 3′-UTR terminator (191 bp;a, Test). The control construct (b) contained in addition to the 1638-bpγ-zeinpromoter, 62 bp of theγ-zeingene 5′-UTR, and the 10-bp 5′-UTR and signal peptide-encoding sequences (78 bp) of theα-L-iduronidasegene. In this case, the 3′-region was from theNos(nopaline synthase) gene (3′-UTR and transcription termination sequences). (c) Northern blot to detect human α-L-iduronidase (IDUA) transcripts in the transgenic developing maize endosperms. The ~2.2-kb IDUA transcripts were detected in different transgenic lines (top panel 1–8); ribosomal RNAs were stained by ethidium bromide to verify the quantity of RNA loaded (lower panel). UT, untransformed control; 1–7, independent transgenic lines expressing test construct; 8–10, independent transgenic lines expressing control construct. (d) Western blot analysis to detect α-L-iduronidase in transgenic maize seeds. Proteins were extracted from endosperms of T2 developing seeds expressing the test construct (left panel) and from endosperms of T2 mature seeds expressing the control construct (right panel). UT, untransformed control; 1–7, indicate independent transgenic lines. Equal protein (50 μg) was loaded in each lane. Figure 1: Constructs and expression of recombinant human α- L -iduronidase in transgenic maize. Gene constructs for expression in maize seeds and the predicted glycosylation status and subcellular localization of the synthesized protein derived from expression of these constructs ( a , b ). Nos , nopaline synthase ( Nos ) gene 3′-region; SP, signal peptide; 3′-UTR, 3′-untranslated region. The human α- L -iduronidase ( IDUA ) gene was driven by the 1638-bp γ-zein promoter (constructs shown in a , b ). Additional γ-zein gene regulatory sequences flanking the α- L -iduronidase mature coding region included the 71-bp 5′-UTR, the signal peptide-encoding sequences (57 bp) and the 3′-UTR terminator (191 bp; a , Test). The control construct ( b ) contained in addition to the 1638-bp γ-zein promoter, 62 bp of the γ-zein gene 5′-UTR, and the 10-bp 5′-UTR and signal peptide-encoding sequences (78 bp) of the α- L -iduronidase gene. In this case, the 3′-region was from the Nos ( nopaline synthase ) gene (3′-UTR and transcription termination sequences). ( c ) Northern blot to detect human α- L -iduronidase (IDUA) transcripts in the transgenic developing maize endosperms. The ~2.2-kb IDUA transcripts were detected in different transgenic lines (top panel 1–8); ribosomal RNAs were stained by ethidium bromide to verify the quantity of RNA loaded (lower panel). UT, untransformed control; 1–7, independent transgenic lines expressing test construct; 8–10, independent transgenic lines expressing control construct. ( d ) Western blot analysis to detect α- L -iduronidase in transgenic maize seeds. Proteins were extracted from endosperms of T2 developing seeds expressing the test construct (left panel) and from endosperms of T2 mature seeds expressing the control construct (right panel). UT, untransformed control; 1–7, indicate independent transgenic lines. Equal protein (50 μg) was loaded in each lane. Full size image Northern blot analysis showed that the α- L -iduronidase gene was transcribed in developing seeds (18–20 days after pollination, DAP) of independent transgenic lines ( Fig. 1c ), albeit to variable extents. Western blot analysis detected α- L -iduronidase protein in mature or developing T2 seeds of most of the lines ( Fig. 1d ). The highest expressing line for the test construct accumulated α- L -iduronidase in the endosperm at 0.12% total soluble protein (T2 seeds). The estimated yield of α- L -iduronidase for the highest expressing line was ~5.2 mg α- L -iduronidase per kg fresh weight (or ~9.4 mg α- L -iduronidase per kg dry weight) at 20 DAP. The estimated yield of α- L -iduronidase derived from expression of the control construct was lower than that derived from the test construct; amongst the transgenic lines analysed, the maximum was ~0.07% TSP. γ-Zein regulatory sequences target mRNA to protein body–ER To determine whether γ-zein regulatory sequences are sufficient for the localization of α- L -iduronidase mRNAs to the protein body–ER of maize endosperm cells, we examined the distribution of α- L -iduronidase mRNAs in cryosectioned developing maize endosperms using in situ RT–PCR. Confocal microscopy showed that α- L -iduronidase mRNAs of the test lines were co-localized exclusively to the protein body regions, having a distribution similar to that of γ-zein mRNAs. In contrast, α- L -iduronidase mRNAs from the control lines were localized to the protein body and non-protein body (cisternal ER) regions ( Fig. 2 ). These data suggest that mRNAs of α- L -iduronidase with 5′-UTR, signal peptide and 3′-UTR sequences from the γ-zein gene are transported to protein body–ER. 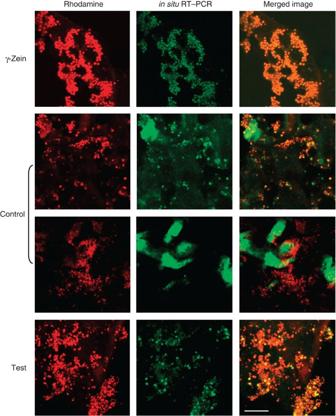Figure 2: Subcellular localization of α-L-iduronidase mRNAs in developing transgenic endosperm sections. Endosperm sections expressing theα-L-iduronidasegene (control and test constructs) were subjected toin situRT–PCR to assess mRNA localization (middle images). ER-derived protein bodies (1 to 2-μm in diameter) were visualized by staining the sections with rhodamine hexyl ester (left images), a dye that preferentially stains the prolamin protein bodies of maize. α-L-Iduronidase mRNAs werein situ-labelled by Oregon Green-dUTP (middle images). In the control sections, α-L-iduronidase mRNAs were seen in both protein body–ER (yellow in the merged image) and in cisternal ER regions (green in the merged image). In contrast, α-L-iduronidase mRNAs derived from the test construct were seen exclusively in the protein body–ER region. Bar, 10 μm. Figure 2: Subcellular localization of α- L -iduronidase mRNAs in developing transgenic endosperm sections. Endosperm sections expressing the α- L -iduronidase gene (control and test constructs) were subjected to in situ RT–PCR to assess mRNA localization (middle images). ER-derived protein bodies (1 to 2-μm in diameter) were visualized by staining the sections with rhodamine hexyl ester (left images), a dye that preferentially stains the prolamin protein bodies of maize. α- L -Iduronidase mRNAs were in situ -labelled by Oregon Green-dUTP (middle images). In the control sections, α- L -iduronidase mRNAs were seen in both protein body–ER (yellow in the merged image) and in cisternal ER regions (green in the merged image). In contrast, α- L -iduronidase mRNAs derived from the test construct were seen exclusively in the protein body–ER region. Bar, 10 μm. Full size image α- L -Iduronidase is targeted to ER-derived protein bodies To investigate whether α- L -iduronidase was targeted to protein bodies within developing maize endosperm cells, immunolocalization studies using transmission electron microscopy (TEM) were conducted. In the ultrathin sections from the control line, there were few 10-nm gold particles (labelled α- L -iduronidase) in ER-derived protein bodies; 10-nm gold particles were predominantly seen in irregular-shaped organelles ( Fig. 3 ; Supplementary Table S1 ). The irregular-shaped organelles were distinguishable from ER-derived protein bodies and are similar to the legumin-type protein storage vacuoles [19] that may originate from a post Golgi process. However, in the sections from the test line, 10-nm gold particles were mainly found in ER-derived protein bodies ( Fig. 3 ; Supplementary Table S1 ). γ-Zein protein was preferentially localized at the periphery of protein bodies (labelled by 5-nm gold particles; arrows), consistent with the reports of others. 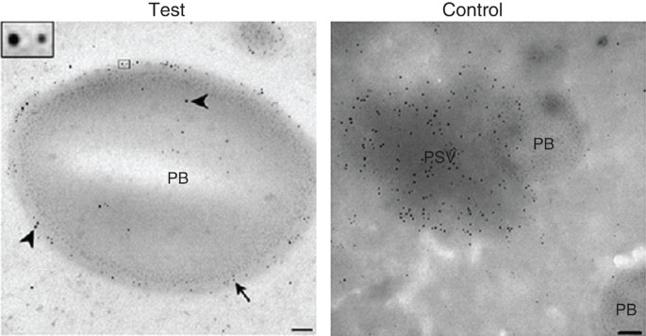Figure 3: Subcellular localization of human α-L-iduronidase protein in developing maize endosperm cells by transmission electron microscopy. Transmission electron microscope images of gold-immunolabelled ultra-thin sections of maize endosperm. α-L-Iduronidase (IDUA) and γ-zein were labelled with 10-nm (arrowheads) and 5-nm (arrows) gold-conjugated secondary antibodies, respectively. Shown are protein bodies (PB) in maize endosperm cells expressing the test construct (left) or control construct (right). PSV=protein storage vacuole. The inset in the left image shows an enlargement of the two sizes of gold particles. Bar=100 nm. Figure 3: Subcellular localization of human α- L -iduronidase protein in developing maize endosperm cells by transmission electron microscopy. Transmission electron microscope images of gold-immunolabelled ultra-thin sections of maize endosperm. α- L -Iduronidase (IDUA) and γ-zein were labelled with 10-nm (arrowheads) and 5-nm (arrows) gold-conjugated secondary antibodies, respectively. Shown are protein bodies (PB) in maize endosperm cells expressing the test construct (left) or control construct (right). PSV=protein storage vacuole. The inset in the left image shows an enlargement of the two sizes of gold particles. Bar=100 nm. Full size image Cell fractionation studies further confirmed the localization of the 'control' and 'test' α- L -iduronidase ( Supplementary Fig. S1 ). These data indicate that cis -localization elements in the γ-zein 5′-UTR, signal peptide-encoding and/or 3′-UTR terminator sequences effectively targeted the α- L -iduronidase RNA molecules to the protein body–ER in developing maize endosperm cells. Furthermore, there was a close relationship between α- L -iduronidase RNA localization and protein localization in the endomembrane system of maize endosperm cells. Recombinant α- L -iduronidase contains high-mannose N-glycans α- L -Iduronidase has six consensus signals for N-linked glycosylation in the ER; these are all utilized in human cells in which the enzyme is targeted to the lysosome via the Golgi complex. In Chinese hamster ovary (CHO) cells hosting production of the recombinant protein, the enzyme is secreted and all six glycosylation sites are used, but the N-glycans themselves display high intrasite heterogeneity [20] . Some of the N-glycans of the mature enzyme remain in a high-mannose form (Asn 372; Asn 415 is mixed high mannose and complex); at least two of the sites are modified to complex forms (Asn 110 and Asn 190); two carry M6P tags (Asn 336 and Asn 451) [20] . The N-glycan profiles of purified α- L -iduronidase of transgenic maize seeds were analysed ( Fig. 4 ; Table 1 ). SDS–polyacrylamide gel electrophoresis (SDS–PAGE) analysis of the purified α- L -iduronidase samples, and the specific activities and yield of recombinant α- L -iduronidase during the purification procedure are shown in Supplementary Fig. S2 and Supplementary Table S2 . As shown, 91.8% of the N-glycan structures detected in the 'test' α- L -iduronidase were of the oligomannosidic type (that is, those containing 1–7 hexose residues in addition to the pentasaccharide N-glycan core) with Man5 being the most abundant (41.1%). The remaining 8.2% were complex/hybrid structures, indicating that some of the human α- L -iduronidase likely transited through the Golgi complex. In contrast, 58.5% of the N-glycans identified in the 'control' α- L -iduronidase belonged to the complex/hybrid type, carrying xylose, fucose or both sugar residues attached to the chitobiose core pentasaccharide. These results further confirm that the 'test' α- L -iduronidase is predominantly localized in ER-derived protein bodies and thereby avoids N-glycan maturation associated with transit through the Golgi complex. The small amounts of recombinant α- L -iduronidase containing the complex N-glycan sugars xylose and/or fucose in the 'test' sample were eliminated by subsequent column chromatography using an anti-horseradish peroxidase affinity column ( Fig. 5 ). 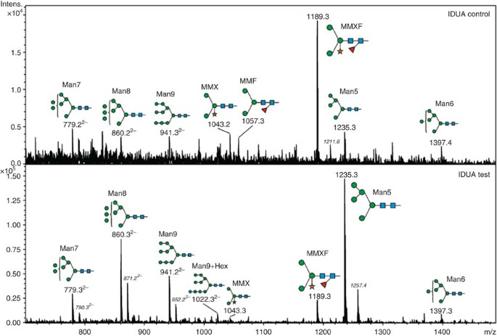Figure 4: N-glycan profiles of maize-derived α-L-iduronidase. Summed MS-spectra of N-glycans from 'control' α-L-iduronidase (IDUA control: top) and 'test' α-L-iduronidase (IDUA test: bottom). In addition to the qualitative N-glycan structure differences, a considerable difference in the signal intensities between the two samples was detected, indicating different amounts of starting material (seeMethods). N-acetylglucosamine (GlcNAc)=blue squares, mannose (M or Man)=green circles, α-1,3-fucose (F)=red triangles, β-1,2-xylose (X)=orange stars. Figure 4: N-glycan profiles of maize-derived α- L -iduronidase. Summed MS-spectra of N-glycans from 'control' α- L -iduronidase (IDUA control: top) and 'test' α- L -iduronidase (IDUA test: bottom). In addition to the qualitative N-glycan structure differences, a considerable difference in the signal intensities between the two samples was detected, indicating different amounts of starting material (see Methods ). N-acetylglucosamine (GlcNAc)=blue squares, mannose (M or Man)=green circles, α-1,3-fucose (F)=red triangles, β-1,2-xylose (X)=orange stars. Full size image Table 1 N-glycans identified in maize-derived α- L -iduronidase. 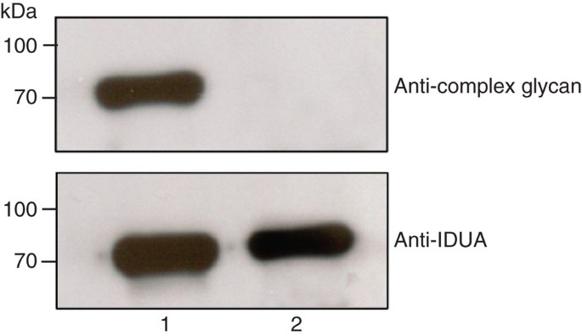Figure 5: Effects of anti-horseradish peroxidase affinity column on the presence of α-L-iduronidase containing plant complex N-glycans. Shows western blot analysis using an antibody specific for plant complex N-glycans as described in theSupplementary Methods. α-L-Iduronidase was purified from transgenic maize seeds expressing the test-construct. Lane 1, 80-ng purified α-L-iduronidase; lane 2, 80 ng α-L-iduronidase after passing through an anti-horseradish peroxidase affinity column. Full size table Figure 5: Effects of anti-horseradish peroxidase affinity column on the presence of α- L -iduronidase containing plant complex N-glycans. Shows western blot analysis using an antibody specific for plant complex N-glycans as described in the Supplementary Methods . α- L -Iduronidase was purified from transgenic maize seeds expressing the test-construct. Lane 1, 80-ng purified α- L -iduronidase; lane 2, 80 ng α- L -iduronidase after passing through an anti-horseradish peroxidase affinity column. Full size image α- L -Iduronidase has high activity and can be phosphorylated Michaelis–Menten kinetics were used to characterize the enzymatic properties of the maize 'test' α- L -iduronidase and the commercial CHO-cell-derived enzyme product, Aldurazyme ( Fig. 6a ; K m and k cat in Supplementary Table S3 ). CHO-iduronidase has a k cat of 3.9 μmoles min −1 mg −1 and a K m of 24 μM; the targeted-maize iduronidase has a k cat of 6.4 μmoles min −1 mg −1 and a K m of 78 μM. In addition, the CHO cell-derived α- L -iduronidase and targeted maize α- L -iduronidase exhibited specific activities of 4.1 and 5.8 μmoles min −1 mg −1 , respectively, when measured at a substrate concentration of 1 mM. 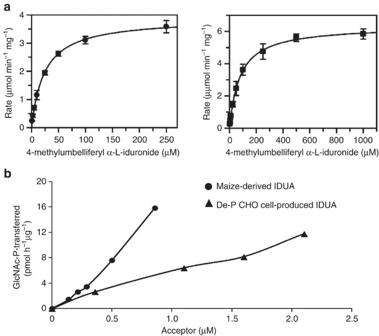Figure 6: Characterization of maize-derived α-L-iduronidase. (a) Michaelis–Menten plots using the fluorescent substrate 4-methylumbelliferyl-α-L-iduronide for CHO cell-produced α-L-iduronidase (Aldurazyme) (left panel) and maize-produced α-L-iduronidase (right panel). The data are the means of three replicate experiments ±s.e. (b) Phosphorylation of maize-produced α-L-iduronidase by the GlcNAc-1-phosphotransferase (α2β2). The graph is based on data from one typical experiment. Dephosphorylated CHO cell-produced α-L-iduronidase served as a control. The activity of the GlcNAc-1-phosphotransferase was expressed as pmoles of [3H]GlcNAc-P transferred per h μg−1of the GlcNAc-1-phosphotransferase. Figure 6: Characterization of maize-derived α- L -iduronidase. ( a ) Michaelis–Menten plots using the fluorescent substrate 4-methylumbelliferyl-α- L -iduronide for CHO cell-produced α- L -iduronidase (Aldurazyme) (left panel) and maize-produced α- L -iduronidase (right panel). The data are the means of three replicate experiments ±s.e. ( b ) Phosphorylation of maize-produced α- L -iduronidase by the GlcNAc-1-phosphotransferase (α 2 β 2 ). The graph is based on data from one typical experiment. Dephosphorylated CHO cell-produced α- L -iduronidase served as a control. The activity of the GlcNAc-1-phosphotransferase was expressed as pmoles of [ 3 H]GlcNAc-P transferred per h μg −1 of the GlcNAc-1-phosphotransferase. Full size image Most lysosomal enzymes including α- L -iduronidase require an M6P tag for efficient uptake/lysosomal delivery in human cells. We investigated whether the phosphorylation of N-glycan terminal mannose residues of the 'test' α- L -iduronidase could be achieved in vitro using recombinant soluble UDP–GlcNAc:lysosomal enzyme N -acetylglucosamine-1-phosphotransferase [21] ( Fig. 6b ). The efficiency of the phosphotransferase is reliant upon its affinity for the target lysosomal hydrolase [22] ; the maize α- L -iduronidase exhibited a K m (0.87±0.1 μM; Supplementary Table S4 ), which is about 25 times less than that of cathepsin D [22] , suggesting that it is an effective substrate for the phosphotransferase. The extent of phosphorylation of a glycoprotein by the phosphotransferase is influenced by the position of the N-glycans relative to the binding site for the phosphotransferase; this modifying enzyme functions best on target lysosomal hydrolases with Man6–Man8 N-glycans [23] , of which the maize α- L -iduronidase has a significant proportion. The k cat value of the maize α- L -iduronidase (0.52±0.18 min −1 ) is comparable to that of the dephosphorylated CHO cell-produced α- L -iduronidase (0.32±0.12 min −1 ; Supplementary Table S4 ). These data show that in vitro phosphorylation is feasible using the plant-derived mannose-terminated recombinant enzyme. We have used a seed-based system towards developing an alternative to the current mammalian cell-based protein production systems. A unique mRNA targeting strategy was used to control the plant-specific N-glycosylation of a complex recombinant human therapeutic enzyme—α- L -iduronidase, a protein possessing six sites for N-glycosylation. Our approach exploits the natural capacity of the endosperm storage tissues of maize seeds to stably accumulate recombinant proteins. The cis mRNA targeting elements provided by sequences of the 27-kDa γ-zein gene successfully mediated the targeting of α- L -iduronidase transcripts and proteins to protein body–ER regions and to ER-derived protein bodies, respectively. Transit of the recombinant protein through the Golgi complex and the consequent undesirable N-glycan maturation was largely avoided. From the point of view of recombinant protein production platforms, the current production systems for ERT and the resultant enzyme therapeutics have some drawbacks that justify an examination of potential alternatives. The prices set for ERT are exceedingly high, placing a considerable burden on health-care budgets and blocking access to ERT in underprivileged countries, and there is little commercial interest towards developing ERT for the ultra-rare LSDs. Safety concerns associated with product contamination included the recent and highly publicized viral contamination of the CHO cell cultures at Genzyme Corporation, which resulted in interrupted or dose-reduced treatments, or the initiation of alternative treatments [24] . Perhaps also of importance, there is considerable N-glycan heterogeneity and variability of glycoforms of a recombinant protein depending on the CHO cell culture conditions [25] of possible relevance to immunogenicity issues [26] . Plant- and seed-based systems provide a potential alternative by virtue of a minimal possibility of contamination by human pathogens or prions, and an ability to rapidly increase biomass without the need for expensive fermentation costs [8] . Maize as a host for recombinant protein production has considerable advantages, including the highest biomass yield among seed crops, ease of transformation/scale-up and the availability of strong promoters and other gene-regulatory sequences to facilitate high-level recombinant protein production. Seeds offer a significant advantage in relation to the provision of a stable repository of the human recombinant protein [8] . In our case, the transgenic maize seeds simply need to be placed in cool dry conditions after harvest, and the human recombinant enzyme remains stable. For example, as compared with the specific activity of the purified protein from freshly harvested mature dry seeds, that associated with the seeds stored for 14 months at 4 °C is very similar (5.8 versus 5.1 μmol min −1 mg −1 , respectively). The major costs associated with the seed-based production system are anticipated to be those associated with downstream purification and processing of the recombinant protein. The control of glycosylation is paramount to the ultimate utility of any plant-derived therapeutic; the addition of xylose and/or fucose sugar residues can elicit immunogenic responses in mammals and greatly reduce the efficacy of plant-derived recombinant proteins for pharmaceutical uses [9] . Our unique strategy may permit the synthesis of pharmaceutical and other recombinant proteins containing predominantly high-mannose N-linked glycans; an affinity column step removed the small amounts of recombinant enzyme containing xylose and/or fucose. The use of mRNA localization signals as a strategy for ER retention of plant-synthesized recombinant proteins is also attractive, as it does not require the fusion of mature protein-coding sequences onto the recombinant therapeutic protein. Other plant-based platforms have been developed to control N-glycan maturation. Fusion of the ER retention/retrieval motif KDEL/HDEL or its extended version (for example, SEKDEL) to the C terminus of a recombinant protein has been a widely used strategy to avoid plant-specific N-glycan maturation. In particular, this strategy has been very effective when applied to the plant-based production of antibodies. However, KDEL-tagged α- L -iduronidase produced in Arabidopsis seeds contains predominantly complex and hybrid N-glycans (88%) [15] . RNA interference technology has been employed in plants to silence the expression of the genes encoding α-1,3-fucosyltransferase and β-1,2-xylosyltransferase. Use of this strategy for production of a monoclonal antibody generates the predominant N-glycan species GnGn (GlcNAc 2 Man 3 GlcNAc 2 ), and few or no α-1,3-fucose and β-1,2-xylose residues are detectable on the protein's N-glycans [27] , [28] . Although this strategy addresses problems associated with plant-specific N-glycan maturation in relation to product immunogenicity, its efficiency in some plant hosts is not absolute [8] , [9] , and further, the predominant N-glycan structures are such that the approach is not useful for the production of therapeutics for LSDs in which mannose-terminated N-glycans or M6P tags on the recombinant protein are essential for therapeutic delivery/efficiency. For therapeutic efficacy, the parenterally administered recombinant enzyme must be competent for endocytosis by human cells, followed by intracellular targeting to the lysosome. These receptor-mediated processes are dependent on either the M6P motif or on mannose-terminated N-glycans on the protein. For those lysosomal enzymes (such as α- L -iduronidase and several others) that generally require an M6P tag for efficient targeting/lysosomal delivery to cells other than macrophages, we show that the high-mannose-terminated, plant-derived recombinant enzyme is an effective substrate for the soluble phosphotransferase as a first step. The plant-based platform founded on mRNA targeting could also be used to generate mannosylated therapeutic glycoproteins that specifically target to the mannose-specific cell surface receptors of macrophages and dendritic cells. This is relevant for the production of recombinant glucocerebrosidase for treatment of Gaucher disease, in which successful ERT relies primarily on mannose receptor-mediated uptake, and it would avoid the three-step downstream processing that is currently used to expose core mannoses to generate the commercial CHO cell-derived product. A carrot cell-based system developed by Protalix and Pfizer for production of recombinant glucocerebrosidase has the advantage of avoiding the need for this in vitro enzymatic processing, and the product (Taliglucerase Alfa) has received recent approval by the US Food and Drug Administration for treatment of Gaucher disease. However, the approaches used for production of the carrot glucocerebrosidase would not be suitable for α- L -iduronidase as an MPS I therapeutic in relation to N-glycan status, therapeutic efficacy requirements and potential immunogenicity. Taliglucerase Alfa has extra amino acids on both the N terminus and the C terminus, and the dominant N-glycans contain xylose and/or fucose residues [29] . Our results provide proof of concept for generating recombinant proteins with high-mannose N-glycosylation in maize seeds. They represent an advance in the field of plant-made pharmaceuticals in relation to generating non-immunogenic recombinant therapeutic proteins. To develop the platform further for production of M6P-tagged LSD therapeutics, the level of accumulation of the human recombinant protein needs to be improved (0.12% TSP in the present study) to advance efficient purification for scale-up. There are tenable strategies to achieve this, including screening more independent transgenic lines, applying a combination of selection and conventional breeding [30] , [31] , and subjecting the high-expressing immature zygotic maize embryos to a dedifferentiation–regeneration cycle, which acts to reset the epigenetic status of the transgene [32] . Two sequential in vitro enzymatic steps also need to be achieved to confer the M6P tag on the high-mannose-terminated recombinant protein. For this, two enzymes are required: the GlcNAc-1-phosphotransferase and the 'uncovering enzyme' GlcNAc-1-phosphodiester α-N-acetylglucosaminidase [33] , which removes the covering GlcNAc residue to expose the M6P recognition marker. We have shown that the high-mannose-terminated α- L -iduronidase is an effective substrate for the first step using soluble recombinant GlcNAc-1-phosphotransferase, and work is in progress to achieve the uncovering enzyme step. The therapeutic efficacy of the in vitro processed α- L -iduronidase also needs to be tested in cultured MPS I (deficient) cells and in the MPS I mouse model. In relation to our model and other lysosomal enzymes, the platform to create the human protein with high-mannose N-glycans is particularly advantageous, because the product is in a suitable form (Gaucher disease), or can be subjected to phosphorylation or to emerging alternative modifications for enhanced biodistribution of ERT [34] , [35] , [36] . Towards a more widespread use of the platform to generate other types of protein therapeutics (not just LSD therapeutics), downstream modification to improve the serum half-life of the protein therapeutic may be required. In the past few years, many efforts have been geared towards achieving 'humanized' complex N-glycan modifications in planta and thus allowing for the elaboration of terminal galactose or sialic acid residues onto the recombinant glycoprotein (for example, by transgenic expression of the appropriate mammalian enzymes) [37] , [38] , [39] , [40] . A monoclonal antibody (2G12) is sialylated in Nicotiana benthamiana by transient expression of six mammalian genes encoding various enzymes of the sialic acid biosynthetic pathway, including a cyclic monophosphate–N-acetylneuraminic acid synthetase and a CMP–sialic acid transporter [39] . Likewise, the addition of bisected, triantennary and tetraantennary complex N-glycans has been achieved by the simultaneous expression of human genes encoding various N -acetylglucosaminyltransferases (GnTIII, GnTIV and GnTV) in a glycoengineered N. benthamiana mutant lacking the machinery for plant-specific complex N-glycosylation (that is, the xylosyl and fucosyl transferases) [40] . Although some of these modifications may well improve the serum half-life of a protein therapeutic, notably there are clearly examples where it is advantageous for a therapeutic protein to have a shorter in vivo half-life to avoid cell toxicity or immune responses [41] , [42] , [43] . The present platform is flexible in the sense that it generates a product that is directly amenable to downstream modifications as appropriate. Downstream-phosphorylated human enzymes generated by this plant-based strategy may be part of future LSD therapeutics. Constructs for the expression of human α- L -iduronidase To investigate the potential of targeting the recombinant α- L -iduronidase to protein bodies of maize, the human α- L -iduronidase ( IDUA ) gene [44] (GenBank accession no. M74715 ) was driven by the 1638-bp promoter of the gene encoding 27-kDa γ-zein [45] (GenBank accession no. X53514 ). Additional regulatory sequences flanking the α- L -iduronidase mature coding region in control and test constructs are noted in the text describing Fig. 1a,b . To clone the 5′-UTR, signal peptide-encoding sequences and 3′-UTR terminator of the γ-zein gene, genomic DNA was extracted from maize Hi-II. For cloning of the 5′-UTR and signal peptide-encoding sequences, forward primer 5′-CACAGGCATATGACTAGTGGC-3′ and reverse primer 5′-GGAGGTGGCGCTCGCAGC-3′ were used to PCR-amplify the fragment. For cloning of the 3′-UTR, the forward primer 5′-ACGCGTCGACAGAAACTATGTGCTGTAGTA-3′ and reverse primer 5′-CGGAATTCCCTATTAAAAGGTTAAAACGT-3′ were used. The DNA sequence encoding the γ-zein signal peptide was fused in-frame to the mature coding region of the α- L -iduronidase gene. Constructs were verified by DNA sequencing. Methods for Agrobacterium -mediated maize transformation are noted in the Supplementary Methods section. RNA extraction and northern blot analysis Total RNA was extracted from developing maize seeds using the Qiagen RNAeasy kit (Qiagen Inc., Mississauga, ON, Canada). Ten micrograms of total RNA was loaded into each lane and RNA samples were fractionated on 1.0% agarose formaldehyde gels. Ribosomal RNA was stained by ethidium bromide to verify the quantity of RNA loaded on the gels used for northern blots. Following transfer and fixing of RNA to Hybond-XL nylon membranes (Amersham Life Science, Buckinghamshire, UK), the membranes were hybridized with a 32 P- α- L -iduronidase cDNA probe that had been labelled using the RTS RadPrime DNA Labelling System (Life Technologies, Gaithersburg, MD, USA) and [α- 32 P]-dCTP. Western blot analysis Proteins were extracted from endosperms of developing T2 seeds (20 DAP) or from mature T2 seeds. Fifty micrograms of total soluble protein was fractionated on 10% SDS–PAGE gels and western blot analysis was carried out using the Lumigen TMA-6 detection kit as per the manufacturer's instructions (GE Healthcare UK Limited, Little Chalfont Buckinghamshire, UK) Anti-α- L -iduronidase [46] and anti-γ-zein [47] antibodies were used at dilutions of 1:1,000. T2 seeds were produced by either self-pollination or by crossing with the wild-type maize Hi-II line in cases in which there was male or female sterility. The yield of α- L -iduronidase was estimated by scanning densitometry of western blots that had been generated with protein extracts from five seeds (at 20 DAP) per independent transgenic line. The CHO cell-produced α- L -iduronidase of known concentration was used as a standard. Some western blot analyses were conducted on the purified proteins ( Supplementary Methods ). In situ RT–PCR Developing endosperms from test and control lines were excised from 15 DAP maize seeds. Cryosectioning and fixation were performed as described by Washida et al . [48] . In situ RT–PCR was conducted on cryosections according to Washida et al . [48] with modifications. The RT–PCR reaction included 2 mM MgCl 2 , 0.5 mM MnSO 4 , 20 μM each of dATP, dCTP and dGTP, 10 μM dTTP, 10 μM Oregon Green-dUTP (Molecular Probes, Eugene, OR, USA), 5 mM dithiothreitol, 150 U ml −1 RNase inhibitor (Fermentas Corp., Ottawa, ON, Canada), PCR enhancer, 50 U ml −1 Tth DNA polymerase (Epicentre, Madison, WI, USA) and 0.5 μM of α- L -iduronidase gene-specific primers: 5′-GGCCAGGAGATACATCGGTA-3′ and 5′-CTCCCCAGTGAAGAAGTTGG-3′. Primers for the γ-zein gene were: 5′-TGAGGGTGTTGCTCGTTGCCC-3′ and 5′-CACATCGCCGTCAGTTGCTGC-3′. The sections were covered with the above solution and kept at room temperature for 30 min followed by 60 °C for 30 min. The sections were then subjected to 20–25 amplification cycles (10 cycles for γ-zein) of 94 °C for 1.5 min, 55 °C for 1.5 min, 72 °C for 1.5 min, which was followed by 72 °C for 5 min. After the PCR cycles, the sections were washed and stained with rhodamine B hexyl ester according to Washida et al . [48] , mounted in anti-FADE medium and analysed by confocal microscopy using a Bio-Rad Radiance Plus on an inverted Zeiss Axiovert with DIC optics (Bio-Rad, Missasauga, ON, Canada). TEM immunolocalization of α- L -iduronidase in maize seeds Developing endosperms (15-17 DAP) were fixed with a high-pressure freezer (Bal-Tec HPM 010 High Pressure Freezer, Zurich, Switzerland). Ultrathin sections were acquired using a Leica UltracutT UltraMicrotome (Reichert, Austria). The sections were picked up on 200 mesh nickel grids, and non-specific binding sites were blocked by immersion in blocking buffer (2% normal goat serum in PBS, pH 7.2) for 1–2 h. The sections were then labelled with antibody against α- L -iduronidase (1:20 dilution) for 1 h and rinsed extensively followed by incubation with 10 nm gold-conjugated goat anti-rabbit IgG (whole molecule; 1:100 dilution) for 1 h. After rinsing several times, the sections were labelled with the antibody against γ-zein (1:50) and 5 nm gold-conjugated goat anti-rabbit Fab′ fragments (1:100), sequentially. All the antibodies were diluted in 2% goat serum-blocking solution. The grids were observed under a TEM Model Hitachi-80 (Hitachi, Tokyo, Japan). Determination of N-glycan profiles of α- L -iduronidase Purified 'test' α- L -iduronidase or 'control' α- L -iduronidase (~4 μg) was resolved by 10% SDS–PAGE, and the α- L -iduronidase protein bands were recovered from the gel. N-glycans were released from tryptic peptides obtained after in-gel digestion as described by Kolarich and Altmann [49] , but graphitized carbon liquid chromatography MS/MS (carbon LC-MS/MS) was used for N-glycan analysis [50] . Therefore, the released N-glycans were reduced and desalted before analysis as described previously [50] . An aliquot of the released and reduced glycans was analysed by carbon LC-MS/MS using an Agilent 1100 capillary LC and an Agilent ion trap for detection using a Thermo Hypercarb column (180 μm ID×100 mm length). N-glycans were analysed using negative mode according to Wilson et al . [50] . Oligosaccharide structures were assigned based on mass, MS/MS spectra and on the knowledge about plant N-glycosylation [51] . The relative N-glycan distribution was calculated from the signal intensities of the monoisotopic m/z signals in the combined MS spectrum, which was summed over the entire range where the N-glycans are eluting. If the singly and doubly charged signal was detected, both signals were taken into account. The summed MS spectra of N-glycans showed a considerable difference in the signal intensities between the two samples detected, indicating different amounts of starting material. Equal amounts of test and control α- L -iduronidase were loaded onto the gels for fractionation before N-glycan purification, reduction/desalting and analysis (see above). However, for some unknown reason, some of the protein from the control α- L -iduronidase sample appeared to have precipitated and remained stacked in the wells of the SDS–PAGE gel after electrophoresis. Small N-glycans consisting of a single GlcNAc residue cannot be released by enzymatic treatment and can only be detected on the glycopeptides; this was not investigated in the present study. Modification of α- L -iduronidase by GlcNAc-phosphotransferase For in vitro phosphorylation of maize-derived α- L -iduronidase, the recombinant α 2 β 2 GlcNAc-1-phosphotransferase (0.15 μg) was added to the reaction mixtures containing various concentrations of maize-derived α- L -iduronidase in 50 mM Tris-HCl, pH 7.4, 10 mM MgCl 2 , 10 mM MnCl 2 , 75 μM UDP-[ 3 H]GlcNAc (1 μCi) and 2 mg ml −1 bovine serum albumin in a final volume of 50 μl. Dephosphorylated CHO cell-produced α- L -iduronidase served as a control. The assay was carried out as described by Qian et al . [22] . Apparent K m and k cat values were generated from double-reciprocal plots using a least square approximation for the best-fit line. The K m and k cat values ( Supplementary Table S4 ) are the means of three separate determinations. The graph of the activity of GlcNAc-1-phosphotransferase (α 2 β 2 ) towards α- L -iduronidase ( Fig. 6b ) was based on data from one typical experiment. CHO cell-produced α- L -iduronidase was dephosphorylated using calf intestinal phosphatase (New England Biolabs Ltd., Pickering, ON, Canada) at 0.5 unit μg −1 Aldurazyme overnight at room temperature. Dephosphorylated CHO cell-produced α- L -iduronidase was dialyzed at 4 °C overnight in a buffer containing 20 mM Tris-HCl, pH 7.4, 10 mM MgCl 2 , 150 mM NaCl and 0.05% Triton X-100. How to cite this article : He, X. et al . Production of α- L -iduronidase in maize for the potential treatment of a human lysosomal storage disease. Nat. Commun . 3:1062 doi: 10.1038/ncomms2070 (2012).